An ultracompact X-ray source based on a laser-plasma undulator The capability of plasmas to sustain ultrahigh electric fields has attracted considerable interest over the last decades and has given rise to laser-plasma engineering. Today, plasmas are commonly used for accelerating and collimating relativistic electrons, or to manipulate intense laser pulses. Here we propose an ultracompact plasma undulator that combines plasma technology and nanoengineering. When coupled with a laser-plasma accelerator, this undulator constitutes a millimetre-sized synchrotron radiation source of X-rays. The undulator consists of an array of nanowires, which are ionized by the laser pulse exiting from the accelerator. The strong charge-separation field, arising around the wires, efficiently wiggles the laser-accelerated electrons. We demonstrate that this system can produce bright, collimated and tunable beams of photons with 10–100 keV energies. This concept opens a path towards a new generation of compact synchrotron sources based on nanostructured plasmas. Today’s brightest X-ray beams are generated by synchrotron radiation (SR) sources [1] , [2] , [3] . In industry, biology and basic research, this radiation is used for ultrafast transient imaging with angstrom resolution. SR is produced by electrons, which are accelerated to relativistic energies and injected into a spatially modulated field. The electrons oscillate in this field and radiate light at a frequency, which is the frequency of their own oscillations up-shifted by a factor , where γ e = ε e / m e c 2 is the Lorentz factor of an electron with an energy ε e . In conventional SR sources, the undulating field is produced by a periodic structure of permanent magnets. For efficient X-ray generation, metre-long magnetic undulators with a period of 1–10 centimetres are required. The relativistic electron beams are typically provided by large-scale accelerator facilities. Laser-plasma accelerator (LPA) constitutes an alternative to traditional radiofrequency linear accelerators in the production of the energetic electron beams [4] , [5] , [6] , [7] , [8] . They have the potential to reduce the size of electron accelerators down to few millimetres. Indeed, as an ionized medium, plasma can withstand much higher fields than the cavity walls in conventional accelerators, which are subject to electrical breakdown. Besides particle acceleration, laser-plasma technology can be used, for instance, in plasma mirrors [9] , to manipulate high-intensity laser pulses [10] , or to collimate relativistic electrons [11] . In LPA, an ultrashort laser pulse is focused into a gas medium. The laser ionizes the gas and drives a copropagating plasma wave, in which electrons can be trapped and accelerated. State-of-the-art LPA delivers reproducible and quasi-monoenergetic electron beams with energies of hundreds of MeVs [8] , and records values that exceed 3 GeV [12] . The electron beams have micrometre source sizes and carry electron currents of tens of kilo-Amperes. This extremely high electron flux suggests that LPA can produce very bright SR that opens the path for a compact free electron laser [13] . SR sources based on a combination of LPA and magnetic undulators have recently been demonstrated for visible light [14] and soft X-ray [15] emission. These experiments were performed with metre-scale magnetic undulators that were placed tens of centimetres after the exit of the accelerator. However, as the divergence of the electron beam in LPA is typically of a few milliradians, the electron flux can be reduced by four orders of magnitude after propagation of 10 cm. This rapid decrease in the electron flux strongly limits the brightness of SR sources based on LPA and magnetic undulators and has hindered the development of such sources. In this letter, we present a SR source, which combines laser-plasma engineering and nano-structured targets. The key new element of the proposed scheme is the use of a laser-plasma undulator instead of a magnetic undulator. The undulator consists of an array of cylindrical nanowires arranged in a checkerboard pattern and oriented perpendicularly to the direction of laser propagation. When ionized and heated by the laser field, the wires generate a strong electric field that bends the trajectories of the incoming relativistic electrons. Importantly, the wavelength of this undulator can be as small as a few micrometres. This makes the overall interaction length remarkably short and allows to take advantage of the high electron flux of LPA before it is reduced by the natural divergence of the beam. Principles of the laser-plasma undulator The overall scheme of the proposed light source is presented in Fig. 1 . We consider a 30-fs pulse from a TW-class laser focused into an supersonic gas jet. The laser ionizes the gas and drives a plasma wave in its wake. Some of the electrons of the plasma are trapped in this wave and are accelerated up to a few hundreds of MeV. At the exit of the accelerator, the laser pulse and the electron beam propagate through a millimetre-scale vacuum space before entering the undulator region. The wires have a typical diameter of few hundreds of nanometres, and are 10–20 μm long. 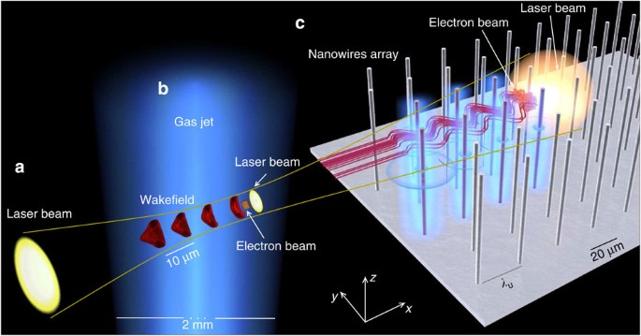Figure 1: Conceptual design of the laser-plasma SR source. (a) An intense laser pulse (yellow) is focused in a gas jet. (b) The laser pulse propagates through the gas jet, trapping and accelerating an electron bunch in its wake. (c) The laser pulse ionizes the nanowires, heats their electrons and creates an electrostatic field (in blue). The trailing electron bunch wiggles in this field (red trajectories). Figure 1: Conceptual design of the laser-plasma SR source. ( a ) An intense laser pulse (yellow) is focused in a gas jet. ( b ) The laser pulse propagates through the gas jet, trapping and accelerating an electron bunch in its wake. ( c ) The laser pulse ionizes the nanowires, heats their electrons and creates an electrostatic field (in blue). The trailing electron bunch wiggles in this field (red trajectories). Full size image The wire spacing along the electron propagation defines the undulator period λ u . The transverse wire spacing determines the amplitude of the wiggling field, and thus the ability of the undulator to deviate the propagating electrons. In SR science, this ability is characterized by the undulator strength parameter K . This parameter can be defined as the amplitude of the oscillations of the particles’ normalized transverse momentum. The strength of an ideal magnetic undulator depends only on the amplitude of the undulator field B 0 and on its period, and is given by the relation K = eB 0 λ u /(2 πm e c ). In the nanowire undulator, the wiggling field is strongly inhomogeneous, and each particle oscillates with different amplitude. In this case, one should consider the oscillations of individual particles to define the averaged K . In terms of radiation produced, the strength parameter separates the undulator K ≲ 1 and wiggler K >>1 emission regimes [16] . In the undulator regime, electrons emit photons in a narrow energy band around the fundamental wavelength , while in the wiggler regime, they emit a broadband spectrum. The analysis of the operation of a laser-plasma undulator can be divided into three parts: (i) the interaction of the laser field with an individual wire, (ii) the propagation of the laser pulse through the array of wires and (iii) the motion of the electrons in the undulator field and the related emission. i The interaction of a high-power laser pulse with a solid wire leads to the creation of a plasma with a high electron density on the surface of the wire. Such an overcritical plasma is opaque to the laser and thus the laser radiation only penetrates in a nanometre-thin sheath [17] . The electrons in this sheath are heated by the laser field in a process that strongly depends on the laser polarization. In particular, for a laser wave polarized perpendicularly to the wire, the electric field has a component normal to the wire surface, which enhances the heating, in a similar way to Brunel absorption [18] . Once the laser pulse has passed the wire, the expansion of the hot electrons produces a strong charge separation field on the wire surface. The field amplitude E 0 is estimated to be of the same order of magnitude as the laser amplitude E las and it can be as high as a few teravolts per metre. The propagation of the laser and electron beams and the generation of space charge fields are shown in Fig. 2 . Over the femtosecond interaction time, the laser, which has an intensity ~10 19 W cm −2 , does not affect the ion core of the wires. The electrostatic field of the ionized wires remains quasi-constant on the timescale of the Coulomb explosion of the ions. For solid density plasmas, this time is typically around a picosecond. For longer times, the wires will be destroyed by Coulomb explosion. 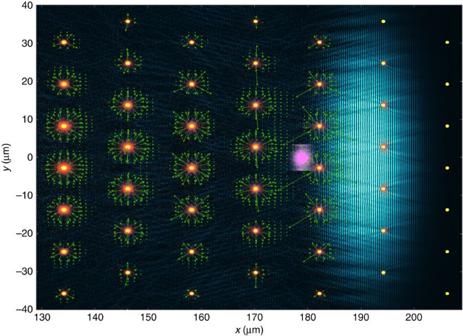Figure 2: Snapshot of a particle-in-cell simulation of the laser-plasma undulator. The laser, which propagates from left to right, and the scattered electromagnetic waves are shown in blue. The relativistic electron beam that follows the laser is represented in pink, the ions and the electrons of the wires are shown in yellow and orange, respectively. The green vectors represent the electric field generated by the plasma wires. In this simulation, the parameters fromTable 1are used. Figure 2: Snapshot of a particle-in-cell simulation of the laser-plasma undulator. The laser, which propagates from left to right, and the scattered electromagnetic waves are shown in blue. The relativistic electron beam that follows the laser is represented in pink, the ions and the electrons of the wires are shown in yellow and orange, respectively. The green vectors represent the electric field generated by the plasma wires. In this simulation, the parameters from Table 1 are used. Full size image ii The energy lost by the laser in the interaction with each wire is either absorbed by hot electrons or carried away by the diffracted electromagnetic wave. A detailed analysis indicates that for the typical parameters presented in Table 1 , diffraction losses dominate over absorption. More precisely, the cylindrical electromagnetic wave that is reflected by the plasma wire carries a fraction of the total laser power. As the laser propagates through the array of wires, the diffraction losses lead to an exponential depletion of the laser intensity with the propagation distance I las ( x ) ∝ exp(− x / l loss ). The characteristic length of energy deposition is given by , where is the effective number of ionized wires, which takes into account the lesser value of the laser intensity at the transverse positions of the wires y j . For parameters given in Table 1 , the laser depletion length is estimated as l loss =0.2 mm. Table 1 Design parameters of the source. Full size table iii The wiggling motion of the electrons from the relativistic bunch can be analysed on two scales. On a short timescale, electrons oscillate in the field surrounding the wires, at the frequency c /λ u , while on a long timescale, the electron beam diverges because the mean field (averaged over λ u ) is defocusing. The electron oscillations and hence the corresponding radiation are characterized by the undulator parameter K and the oscillation wavelength λ u . As K is approximately proportional to the laser field amplitude, it decreases exponentially with the propagation distance, with a characteristic length 2 l loss . The initial value of the undulator parameter K 0 depends on the laser energy and undulator geometry; for the parameters in Table 1 , K 0 ≈0.7. In the limit K ≪ 1 (which is verified after a short propagation), the number of emitted photons per electron oscillation is ~2α K 2 , where α ≃ 1/137 is the fine structure constant [16] . Thus, we estimate that, over their full trajectory, each electron produces photons around an energy . It follows that for a beam charge of 50 pC, the radiation consists of 1.8 × 10 7 photons with energies centred around 12, 48 and 107 keV, for electron energies of 200, 400 and 600 MeV, respectively. Numerical modelling In order to validate the proposed scheme and to predict more precisely the radiation features, the laser-plasma undulator was modelled using particle-in-cell simulations (see Methods). We considered a quasi-monoenergetic electron beam having the properties given in Table 1 , which corresponds to state-of-the-art laser-plasma accelerators [19] , [20] , [21] . Moreover, shown in Table 1 are the laser parameters at the entrance of the undulator. To prevent the supersonic gas jet from influencing the nanowires, a distance of 1 mm between the accelerator and the undulator was chosen, and the drift of the electrons in this vaccuum space was self-consistently taken into account. The interaction of the laser and electron beams with a 14-line undulator was modelled in the two-dimensional (2D) plane ( x , y ). The two characteristic scales of the electron motion are highlighted in Fig. 3 . 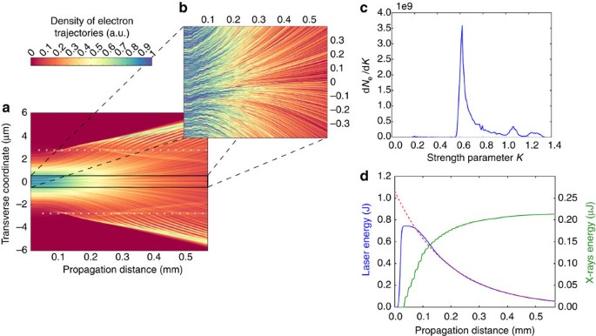Figure 3: Electron and laser propagation in a laser-plasma undulator. (a) Electron trajectories in the undulator, obtained from a 2D PIC simulation. The colour scale indicates the electron density. Propagation and transverse distances are measured in millimetres and micrometres, respectively, and the white markers indicate the positions of the wires. (b) Magnified view of the central part ofa. (c) Distribution of the undulator parameterK, calculated from individual trajectories. (d) Evolution of the total emitted energy (green curve), and the total laser energy in the PIC simulation (blue curve) compared with our modelIlas(x)∝exp(−x/lloss) withlloss=0.2 mm (red dashed line). Figure 3a shows the increase in the electron beam divergence because of the mean transverse field, while Fig. 3b reveals the electron oscillations. The undulator parameter K of each individual particles was calculated from their trajectories over a distance l loss . The distribution of K is shown in Fig. 3c and it exhibits a peak around K =0.6, with an average undulator parameter ‹ K ›=0.73. Simulations also confirm the exponential depletion of the laser (see Fig. 3d ). The predicted depletion length l loss =0.2 mm is in a very good agreement with the simulation, which confirms that the laser energy losses are mainly because of the diffraction by the wires. As the undulator parameter is approximately proportional to the square root of the laser intensity, the number of emitted photons per period varies roughly as the laser energy. It follows that the emission becomes negligible after a propagation exceeding ~3 l loss =0.6 mm. Figure 3: Electron and laser propagation in a laser-plasma undulator. ( a ) Electron trajectories in the undulator, obtained from a 2D PIC simulation. The colour scale indicates the electron density. Propagation and transverse distances are measured in millimetres and micrometres, respectively, and the white markers indicate the positions of the wires. ( b ) Magnified view of the central part of a . ( c ) Distribution of the undulator parameter K , calculated from individual trajectories. ( d ) Evolution of the total emitted energy (green curve), and the total laser energy in the PIC simulation (blue curve) compared with our model I las ( x ) ∝ exp(− x / l loss ) with l loss =0.2 mm (red dashed line). Full size image The SR of an individual electron is emitted in the direction of the electron’s velocity, and within a cone of angle . Therefore, the total radiation emitted by the electron bunch has a minimum angular spread of but may have a larger spread if the divergence of the bunch exceeds . The energy radiated per unit of photon energy and solid angle ∂ 2 ε /∂ ω ∂ Ω is calculated from the Liénard–Wiechert fields. 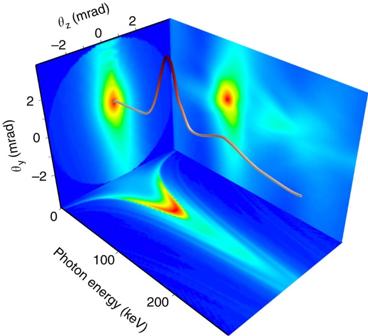Figure 4: Angular-spectral distribution of the produced X-rays. Maps of the emission energy distributions ∂2ε/∂ω∂Ωin the planesy=0 (horizontal plane) andz=0 (right vertical plane), and energy integrated angular distribution (left vertical plane). The angleθyis angular distance along theyaxis, whileθzis that along thezaxis. The curve represents the on-axis spectral distribution. The calculation was performed for 600 MeV electrons. Figure 4 shows the maps of this distribution, in the case of 600 MeV electrons, in the y =0 and z =0 planes (see Fig. 1 for the orientation of these axes), and the angular distribution summed over the photon energy. The angular sizes of the source are Δ θ y =2.3 mrad and Δθ z =0.95 mrad. In the y =0 plane, the photon energy is observed to be distributed around , which is typical for planar undulators. The distribution in the z =0 plane is stretched and flattened because of the growth of the electron beam divergence, which is induced by the undulator-averaged transverse field. In addition, shown in Fig. 4 is the on-axis spectral distribution (red curve). In agreement with the model, the 50 pC electron bunch generates 2.4 × 10 7 photons in a 33% energy-band (full width at half maximum) centred ~100 keV. The total energy of the X-ray beam in this case is 0.18 μJ and its peak brightness is 4.5 × 10 23 photons s −1 mm −2 mrad −2 per 0.1%bandwidth. Figure 4: Angular-spectral distribution of the produced X-rays. Maps of the emission energy distributions ∂ 2 ε /∂ ω ∂ Ω in the planes y =0 (horizontal plane) and z =0 (right vertical plane), and energy integrated angular distribution (left vertical plane). The angle θ y is angular distance along the y axis, while θ z is that along the z axis. The curve represents the on-axis spectral distribution. The calculation was performed for 600 MeV electrons. Full size image Both the photon energy and the source power increase as ; they can therefore be tuned by varying the electron energy. This is demonstrated in Fig. 5 , where the X-ray peak energy is observed to rise from 12 to 106 keV when the electron energy is increased from 200 to 600 MeV. The relative bandwidth of the emitted spectrum remains constant. This shows that quasi-monoenergetic X-rays can be produced in a wide range of wavelengths. 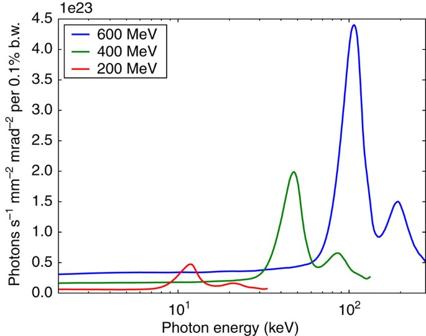Figure 5: On-axis X-ray spectra calculated for different electron energies. Spectral distribution of the source brightness is calculated along the propagation direction for average electron energies of 200 MeV (red curve), 400 MeV (green curve) and 600 MeV (blue curve). Figure 5: On-axis X-ray spectra calculated for different electron energies. Spectral distribution of the source brightness is calculated along the propagation direction for average electron energies of 200 MeV (red curve), 400 MeV (green curve) and 600 MeV (blue curve). Full size image We have presented a new approach that drastically reduces the size, and cost of conventional undulators, and that takes full advantage of the high-flux electron beams produced in laser-plasma accelerators. This laser-plasma undulator consists of an array of periodically assembled nanowires that are ionized by the laser pulse exiting from a laser-plasma accelerator, creating a periodic electric field structure that efficiently operates as an electrostatic undulator. We have shown that this approach can produce bright, polarized and quasi-monoenergetic femtosecond X-ray beams with adjustable energies in the range 10–100 keV and a peak brightness of the order of 10 23 photon s −1 mm −2 mrad −2 per 0.1% bandwidth, using commercially available laser systems. The source properties could be further improved, for example, by reducing the growth of the divergence inside the undulator. Possible improvements include the design of more complex wire patterns, with uneven spacings, variable wire diameters or wire densities. The use of the nanostructured undulator for coherent amplification of X-rays can also lead to the development of an ultracompact X-ray-free electron laser. Moreover, nanostructured laser-plasma devices can be also used to manipulate relativistic particle beams in various ways (for example, wiggling, collimating and focusing). We anticipate that this new approach will open the path for many innovations at the interface between nanoengineering and high-intensity lasers. Numerical modelling of the laser-plasma undulator The formation of the plasma undulator by the laser and the motion of the trailing electrons are studied with the PIC code CALDER 2D [22] . The nanowires are modelled in two dimensions as circles with a radius of 200 nm. They consist of initially neutral atoms of silicon with a density of 5 × 10 22 cm −3 . Ionization is accounted for by using the model of Yudin–Ivanov [23] , [24] . The undulator includes 14 lines of 25 wires (350 wires in total) with transverse spacing 5.5 μm (period 11 μm) and undulator period λ u =24 μm. The moving-window technique is used to study the propagation of the laser and electron beams over a millimetre (the moving simulation box is 46 μm × 70 μm). The spatial resolution is 5 nm. Velocities and positions of the relativistic electrons are recorded each 0.5 fs. These trajectories are then used to compute the radiation produced. The spectral distribution of emitted light is calculated using the Fourier components of Lienard–Wiechert potentials in the far field: The integral is calculated in a three-dimensional angular-spectral space for each particle. The average incoherent spectrum emitted by one electron is calculated as the average of the spectra emitted by the macroparticles. For the spectrum calculation, 1.5 × 10 4 macroparticles were used. How to cite this article: Andriyash, I. A. et al. An ultracompact X-ray source based on a laser-plasma undulator. Nat. Commun. 5:4736 doi: 10.1038/ncomms5736 (2014).